Structure of a bacterial voltage-gated sodium channel pore reveals mechanisms of opening and closing Voltage-gated sodium channels (VGSCs) are composed of two domains, the pore domain that provides the transmembrane pathway for the flow of ions, and the voltage-sensor (VS) domain that is responsible for voltage-mediated gating of the pore. Sodium channels alternate between discrete open and closed states in response to movements of the VS domains, which are transduced via a linker peptide located between the pore and VS domains to a gate located within the pore domain. Prokaryotic VGSCs are homotetramers, with each monomer contributing to both the VS (transmembrane helices S1–S4) and pore (transmembrane helices S5 and S6, and the P1 and P2 helices) domains. Recently, a crystal structure of the NavAb bacterial sodium channel was determined [1] , which was in a hybrid conformation: the pore was closed at its cytoplasmic end, thus having no continuous pathway for ions to cross the membrane, but the VS was in an activated state, which would normally be accompanied by opening of the channel. The S4–S5 linker conformation (between the VS domain and the pore) present in the crystal seems to have inhibited the opening of the channel in the absence of an applied voltage. In this study we created a construct of the pore-only domain of a bacterial homologue of a sodium channel NavMs (Uniprot ID A0L5S6), to produce an open form of a sodium channel. Previous studies have shown that pore-only constructs of prokaryotic sodium channels (consisting of the final two transmembrane segments, S5 and S6) retain both structural and functional properties of the intact channels [2] , [3] . This is because the VS and pore regions of sodium channels (as in the closely related potassium channels) form physically separated domains joined only by the S4–S5 linker peptides [1] . The crystal structure of the pore-only construct of NavMs shows that the channel is in the open conformation, as predicted. Comparisons of this open structure with the structure of the NavAb homologue, in which the activation gate is closed, reveal that the opening is enabled by a rotation around a single bond in the middle of the S6 helix, which results in significant movement of the bottom half of this helix. This movement then creates a large opening at the end of the pore. The internal cavity of the NavMs pore is thus accessible to the cytoplasmic surface, and has an open activation gate of sufficient diameter for hydrated sodium ions to pass through. Its selectivity filter (SF) is very similar to that of the closed form, suggesting that the activation gate is structurally uncoupled from the filter. In addition, its SF includes density that may be attributable to ions and/or water molecules. The transmembrane region includes fenestrations that would enable access of hydrophobic ligands from the membrane to the interior of the channel pore. These fenestrations are considerably larger than those found in the closed form, and thus may have implications for rational drug design. The structure of the open channel The pore-only construct ( Fig. 1 ) of NavMs (PDB accession code 4F4L ) forms stable, folded and active tetrameric channels ( Supplementary Fig. S1 ), which are inhibited by the known channel blocker mibefradil. The tetramer structure ( Fig. 2a ) consists of eight transmembrane helical segments, two per monomer, which form a funnel-shaped bundle. Each of the four monomers in the NavMs tetramer has a slightly different conformation, including the extent of order at both the carboxy- and amino-terminal (C- and N-terminal) ends of the molecule, as well as the angle of bend in the middle of the S6 helix (see discussion below). The cavity through the centre of the channel is formed primarily by the C-terminal S6 transmembrane helices from each of the four monomers (S6 is blue in Fig. 2a , although for clarity only one of the monomers in the tetramer is coloured), with the P1 and P2 helices (green and yellow, respectively), and the SF (red) lining the extracellular half of the pore. The S5 helices (magenta) form the external surface of the bundle. This surface, which would be in contact with the lipid bilayer in both the pore and the intact channel, is almost entirely hydrophobic ( Fig. 2b ). Both the cytoplasmic and extracellular mouths of the pore ( Fig. 2c ) and the entire length of the central cavity have negatively charged surfaces ( Fig. 2d ), compatible with a channel that accommodates and translocates sodium cations. 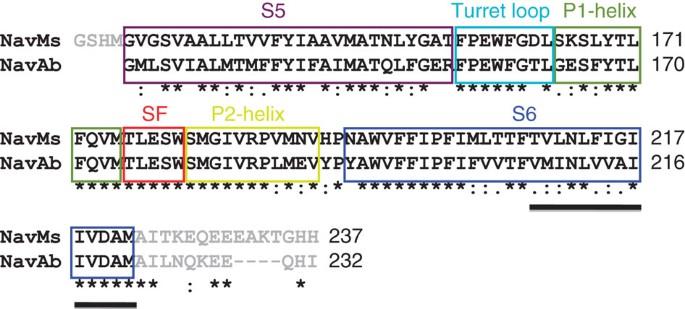Figure 1: Sequence alignment of the NavMs pore construct and the equivalent region of NavAb. Alignments are based on their respective crystal structures, with coloured boxes indicating the locations of the S5 and S6 transmembrane segments (magenta and blue, respectively), the turret loop (cyan), the P1- and P2-helix regions (green and yellow, respectively), the SF (red) and the beginning of the C-terminal domain (the latter, with residue names indicated in grey, is not visible in either of the crystal structures). The black underlined region indicates where the deviation between the S6 helices in the open and closed forms occurs. Figure 1: Sequence alignment of the NavMs pore construct and the equivalent region of NavAb. Alignments are based on their respective crystal structures, with coloured boxes indicating the locations of the S5 and S6 transmembrane segments (magenta and blue, respectively), the turret loop (cyan), the P1- and P2-helix regions (green and yellow, respectively), the SF (red) and the beginning of the C-terminal domain (the latter, with residue names indicated in grey, is not visible in either of the crystal structures). The black underlined region indicates where the deviation between the S6 helices in the open and closed forms occurs. 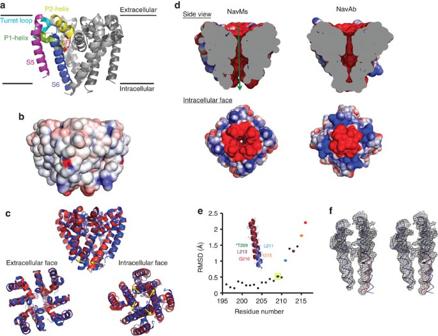Figure 2: Crystal structure of the NavMs pore. (a) The crystal structure of the NavMs pore depicted in ribbon representation13. The regions in one of the four monomers are coloured according to the scheme inFig. 1(blue for the S6 helix, magenta for the S5 helix, green for P1, yellow for P2 and red for the SF), with the other three monomers depicted in grey for clarity. (b) Electrostatic representation of the NavMs pore (from the membrane normal direction), showing that the entire surface is very hydrophobic. (c) Overlaid structures of the NavMs (red) and NavAb (blue) pores depicted in ribbon representations, showing that they are very similar in all regions except the C-terminal end of S6 (closest to the intracellular surface), where they deviate significantly. The directions of the motions are indicated by the yellow arrows. A video morphing between the open and closed structures is included asSupplementary Movie 1. (d) Comparison of the electrostatic surfaces14of the NavMs symmetric pore model (based on a tetramer constructed from the most bent monomer) and the NavAb pore, viewed along the membrane normal and sliced through the middle of the tetramer (top) and from the cytoplasmic surface (bottom). (e) Plot of residue number versus RMSD (root mean square deviation) differences between NavMs (chain A) and NavAb (chain A)Cαpositions in the S6 helix, showing that the major differences occur starting at residue Thr209 (indicated by the yellow box). The colours of the names of the residues identified on the model are reflected in the colour of the points on the plot. (f) Stereo electron density map (2Fo–Fc, 1 σ-contour) of the open-channel conformation (red) backbone atoms overlaid on the closed-channel conformation backbone atoms (blue), which clearly shows the deviation of the structures at the bottom of the S6 helix. Full size image Figure 2: Crystal structure of the NavMs pore. ( a ) The crystal structure of the NavMs pore depicted in ribbon representation [13] . The regions in one of the four monomers are coloured according to the scheme in Fig. 1 (blue for the S6 helix, magenta for the S5 helix, green for P1, yellow for P2 and red for the SF), with the other three monomers depicted in grey for clarity. ( b ) Electrostatic representation of the NavMs pore (from the membrane normal direction), showing that the entire surface is very hydrophobic. ( c ) Overlaid structures of the NavMs (red) and NavAb (blue) pores depicted in ribbon representations, showing that they are very similar in all regions except the C-terminal end of S6 (closest to the intracellular surface), where they deviate significantly. The directions of the motions are indicated by the yellow arrows. A video morphing between the open and closed structures is included as Supplementary Movie 1 . ( d ) Comparison of the electrostatic surfaces [14] of the NavMs symmetric pore model (based on a tetramer constructed from the most bent monomer) and the NavAb pore, viewed along the membrane normal and sliced through the middle of the tetramer (top) and from the cytoplasmic surface (bottom). ( e ) Plot of residue number versus RMSD (root mean square deviation) differences between NavMs (chain A) and NavAb (chain A) C α positions in the S6 helix, showing that the major differences occur starting at residue Thr209 (indicated by the yellow box). The colours of the names of the residues identified on the model are reflected in the colour of the points on the plot. ( f ) Stereo electron density map (2Fo–Fc, 1 σ-contour) of the open-channel conformation (red) backbone atoms overlaid on the closed-channel conformation backbone atoms (blue), which clearly shows the deviation of the structures at the bottom of the S6 helix. Full size image Differences between open- and closed-channel structures Because of the high-sequence identity (67%) of the pore regions of NavMs (residues 131–222) and NavAb (residues 130–221) ( Fig. 1 ), direct comparisons of the closed- (NavAb) and open- (NavMs) transmembrane pathways are possible. The most striking difference between the two structures is in the cytoplasmic half of the molecule ( Fig. 2c ); the cavity in the open form is fully accessible to the aqueous solution along its entire length, whereas in the closed form the cytoplasmic ends of the four monomers are in contact with each other, and there is no access from the cavity to the cytoplasm. The quaternary structural differences result from changes in the organization of the helical segments within each monomer. Although the tertiary arrangements of the helices in the two structures are considerably different, their S5 and S6 transmembrane segments have nearly identical secondary structures ( Fig. 2c ; Supplementary Fig. S2 ). Although the channels are from two different species, and one was crystallized from lipid bicelles and the other from detergent micelles, the three-dimensional structures of the S5 and P-helices, and the N-terminal ends of the S6 helices are very similar in both structures. However, the open and closed structures diverge starting at Thr209 (residue numbering based on the NavMs sequence; Thr84 based on the numbering for the pore in the PDB file 4F4L) in the middle of the S6 helix ( Fig. 1 , black underline), where the open-channel monomer splays outward ( Fig. 2f ), resulting from a modest rotation (~25°) about its ψ -bond that does not disrupt the helical secondary structure ( Supplementary Fig. S2 ), but this produces a bend that does alter the direction of the C-terminal end of the S6 helix considerably. Propagation of this small movement results in a >2.5 Å displacement of the C α atoms at the bottom of one of the S6 segments ( Fig. 2e ), which when part of a tetramer, would result in an aperture in the activation gate with a diameter >8 Å ( Fig. 3a ), easily sufficient for a hydrated sodium ion (roughly 7.8 Å in diameter) to pass through. This produces a continuous open pathway through the centre of the pore ( Figs 2d and 3a ). In contrast, in the NavAb structure the channel becomes too narrow at Ile217 to allow even a dehydrated sodium ion to pass through ( Figs 2d and 3a ). 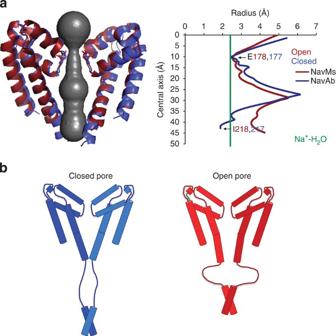Figure 3: Features of the NavMs pore open-channel structure. (a) Left: the accessible inner surface15(in grey) of the NavMs symmetric pore model, showing that there is a continuous pathway from the extracellular to the cytoplasmic surface of the membrane, which is of sufficient size to enable the passage of a fully hydrated sodium ion (except around the SF, where only a hemi-hydrated ion will fit). In this figure the NavMs (red) and NavAb (blue) structures are overlaid as ribbon diagrams. Right: plot of channel radius versus distance along the channel direction for the open NavMs (red) and closed NavAb (blue) structures, showing that in the extracellular half (including the SF and the central cavity), the diameters of the open and closed forms are nearly identical, but that in the region of the activation gate there is a substantial difference in the diameter of the cavity of the open versus closed forms. (b) Schematic model for the opening and closing of bacterial sodium channels, showing changes in the orientations of the bottom half of the S6 helices and the compensating changes required in the disordered regions of the C-terminal domain. Note only two monomers are shown for clarity. Figure 3: Features of the NavMs pore open-channel structure. ( a ) Left: the accessible inner surface [15] (in grey) of the NavMs symmetric pore model, showing that there is a continuous pathway from the extracellular to the cytoplasmic surface of the membrane, which is of sufficient size to enable the passage of a fully hydrated sodium ion (except around the SF, where only a hemi-hydrated ion will fit). In this figure the NavMs (red) and NavAb (blue) structures are overlaid as ribbon diagrams. Right: plot of channel radius versus distance along the channel direction for the open NavMs (red) and closed NavAb (blue) structures, showing that in the extracellular half (including the SF and the central cavity), the diameters of the open and closed forms are nearly identical, but that in the region of the activation gate there is a substantial difference in the diameter of the cavity of the open versus closed forms. ( b ) Schematic model for the opening and closing of bacterial sodium channels, showing changes in the orientations of the bottom half of the S6 helices and the compensating changes required in the disordered regions of the C-terminal domain. Note only two monomers are shown for clarity. Full size image Despite the significant movement of the S6 segments, there is little apparent displacement of the S5 helices that surround the S6 pore ( Fig. 2c ). A movement of only ~1 Å at the N-terminal Ser133 of the S5 helix is required to accommodate the movement of the S6 segments. Consequently, in the full-length channel, opening could be accomplished with a relatively minor change in the position of the S4–S5 linker region from its position in the NavAb structure ( Fig. 4 ). 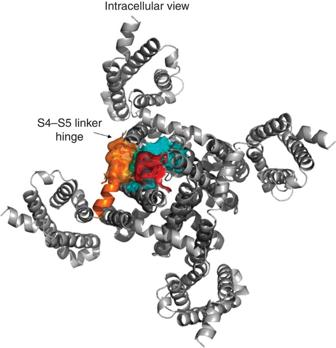Figure 4: Linker movement required to open the pore. Overlay showing the residues (in space-filling representation) involved in potential clashes at the end of the open NavMs (red) with those in the S4–S5 linker hinge region (yellow) of the closed NavAb form (blue). This suggests that in the open form of the full-length NavMs channel, the N-terminal end of S5 and the linker must be in a slightly different position from that present in the NavAb closed structure. Figure 4: Linker movement required to open the pore. Overlay showing the residues (in space-filling representation) involved in potential clashes at the end of the open NavMs (red) with those in the S4–S5 linker hinge region (yellow) of the closed NavAb form (blue). This suggests that in the open form of the full-length NavMs channel, the N-terminal end of S5 and the linker must be in a slightly different position from that present in the NavAb closed structure. Full size image A novel opening/closing mechanism On the basis of the sequence ( Supplementary Fig. S3 ) of the first bacterial VGSC identified [4] (NaChBac), it was proposed [5] that a glycine (residue 219) in the middle of the S6 helix might act as a flexible hinge for the opening and closing of the pore. This idea was partially supported by mutagenesis studies that dramatically modified but did not abolish gating [5] , [6] , and by the observation that replacement of the glycine with a more conformationally constraining residue (that is, serine) [7] resulted in increased thermal stability of the protein. However, glycines are not found at equivalent positions in many of the more recently identified homologues, including NavMs and NavAb ( Supplementary Fig. S3 ), although the threonine at which S6 helix begins to deviate between the open state and the closed state in the crystal structures is only one helical turn away from that glycine position. On the basis of the NavAb crystal structure, it was proposed [1] that opening and closing of the pore would involve an iris-like motion of the S5 and S6 helical segments relative to each other, much as had been proposed for the nicotinic acetylcholine receptor and potassium channels. It was suggested that in response to activation of the VS, the linker could move as a hinge, inducing a slight twist at the base of the S5 helix (possibly involving the conserved Pro–Gly at the end of the S4–S5 linker), mediating the opening by a twisting of the helices with a tight coupling between the motions of S5 and S6 helices. However, based on comparisons of the NavMs and NavAb structures, the mechanism would instead seem to be a rotation around the backbone angle of one residue in the middle of S6 helix, which swings that helix away from the central pore, opening up the bottom of the structure, and creating an unrestricted transmembrane pathway for the ions to traverse ( Supplementary Movies 1 and 2 ). Such a motion does not result in significant impinging of the S6 onto the S5 helix, but must be accommodated by a change within the linker-region position ( Fig. 4 ). The NavAb construct included all of the residues in the C-terminal domain, but the C-terminal residues extending beyond the methionine (residue 221) located at the cytoplasmic end of the S6 helix were not resolved in the structure. In this study, NavMs was truncated at His237 ( Fig. 1 ; Supplementary Fig. S3 ) near the middle of the C-terminal domain. The region beyond the end of the equivalent S6 methionine is also not visible in this crystal structure. Thus, neither crystal structure provides a view of any part of the C-terminal domain. However, synchrotron radiation circular dichroism (CD) spectroscopic studies using sequentially truncated constructs of the NaChBac homologue [8] have indicated that its C terminus consists of a distal coiled-coil region of approximately 20 residues preceded by a disordered region of 12 residues adjacent to the C-terminal end of the S6 helix ( Fig. 3b ). All prokaryotic sodium channel sequences identified to date [4] , [8] , [9] , [10] seem to include a similar motif [8] , [11] . The presence of the helical C-terminal domain is not essential for channel formation in NavMs, but it may have a role in stabilizing the tetramer. The proximal unordered region in the C-terminal domain seen in NaChBac and predicted for the other homologues may, however, be critical in enabling the splaying of the ends of S6 helix upon opening, without uncoiling of the distal coiled-coil domain ( Fig. 3b ). Differences in monomer structures within the tetramer In all of the crystal forms of the NavMs pore, which diffracted to better than 4 Å resolution ( Table 1 ), it was observed that the four monomers (which are not related by a crystallographic fourfold) comprising the tetramer are very similar, but they are not identical. One monomer is better ordered at the C-terminal end of S6 helix (chain D), one better ordered at the N-terminal end of S6 helix (chain C), and all have slightly different bend angles at Thr209. The different bend angles arise from different degrees of rotation about the ψ -angle of Thr209 residue (about 25 o in the case of chain A); for all monomers, the resulting φ,ψ -angle combinations for these residues still lie in the helical region of the Ramachandran plot; the rotations produce a change in direction of the polypeptide ( Fig. 2f ). This results in a displacement of the bottom of S6 helix by 2.5 Å (chain A; Fig. 2e ). Displacements are present in the other three monomers, but to lesser degrees. To demonstrate the maximal extent of opening of the pore, we produced a symmetric tetramer model based on real-space alignments of the most bent (chain A) monomer with the other three monomer positions, using the S5 and top of S6 helices ( Supplementary Fig. S4 ). In this model, the opening at the cytoplasmic end of the cavity ( Fig. 3a ) was >8 Å, which was well sufficient for the passage of a hydrated sodium ion. Interestingly, in the lower-resolution structures ( Table 1 ) from two different detergents, n-nonyl-β- D -maltopyranoside (NM) and decanoyl- N -hydroxyethylglucamide (HEGA-10), which had not been subjected to the partial dehydration protocol essential for improving the diffraction quality, all of the monomers were very similar to each other, and their backbone ( C α atoms) overlaid most accurately (lowest root mean square deviation) with the most bent chain A of the higher-resolution structure, producing structures that were fully open and essentially identical to the fourfold symmetric model ( Supplementary Fig. S4 ). The flexibility in the Thr209 bend that produces the different monomeric structures may be indicative of the range of intermediate structures that can be adopted during the process of channel opening. Indeed, the asymmetry of structure found within the higher-resolution tetramer is reminiscent of the functional asymmetry of eukaryotic VGSCs, in which one of the four domains (albeit, in this case, they all have different sequences) seems to open before the others [12] . Table 1 Data collection and refinement statistics (molecular replacement). Full size table The SF and fenestrations The SFs in the NavMs and NavAb crystal structures are virtually identical ( Fig. 2c ; Supplementary Fig. S5a ), suggesting that SF size and geometry are fixed whether the pore is open or closed. The signature bacterial VGSC filter sequence (LESWS) is present in both structures, and both structures include the stabilizing framework formed from the adjacent aromatic interactions ( Supplementary Fig. S5a ). Glutamates in the SF provide a binding site that could accommodate a hemi-hydrated sodium ion with a 4.6 Å diameter. The electron-density map of NavMs ( Supplementary Fig. S5b ) in the region of the SF indicates the presence of density that could be attributable to sodium ions, although at the resolution of the present structure we cannot confirm whether it is one or more sodium ions, or water molecules. However, the crystallization procedures contained (and indeed, required) the presence of only sodium cations; hence, the density in the SF is not expected to represent any other type of cation. In contrast, no density is apparent in the SF of the closed NavAb structure. It is notable, however, that the polypeptide backbone and side-chain geometries are very similar for the residues in the open and closed structures in this region, suggesting that the SFs are structurally decoupled from changes to the activation-gate structures. As was seen in the closed NavAb structure, there are lateral windows (designated ‘fenestrations’) in the sides of the structure exposed to the membrane, which are contiguous with the inner cavity of the pore ( Supplementary Fig. S6 ). In the closed form, these openings contain density that has been postulated to arise from acyl chains of lipid molecules, but in the open form no such density is evident. This observation is consistent with the proposed nature of the density, as open conformation crystallizations do not contain added lipid molecules. The fenestrations have been proposed [1] to act as entry regions for hydrophobic ligands into the channel interior. However, it was also proposed [1] that they might close in the open state according to the ‘modulated receptor’ model. On the contrary, in the open channel these portals are larger than those seen in the closed structure. This is because the lower end of the S6 helix (in the hinge region) forms part of the boundary of the fenestration ( Supplementary Fig. S6 ), and the splayed S6 helices further open up the sideways entry into the pore. Intriguingly, if the fenestrations are indeed portals that enable entry of ligands, their difference in size between the open and closed states could be exploited in the design of drugs that stabilize the open state. Structure–function relationship of sodium-channel homologues Prokaryotic sodium channels exhibit modest single-channel conductance parameters relative to those of eukaryotic sodium channels [11] ; pore constructs are not voltage-gated, but they do produce single channels [3] . The NavMs channel is a close homologue of NaChBac, which has been clearly demonstrated to be sodium selective. NavMs channels and the pore-only constructs that are described in this work exhibit similar sodium-flux profiles ( Supplementary Fig. S2c ) to NaChBac channels and pores (D’Avanzo et al. , in preparation), as well as to pores and channels of the NavSp [2] homologue; all are inhibited by the channel blocker mibefradil. All bacterial sodium channels exhibit high degrees of sequence identity ( Supplementary Fig. S3 ), and none have amino acid substitutions that would block the open pore as seen in this conformation. However, the NaChBac homologue lacks the relatively conserved methionine at the bottom of S6 helix; instead it (and several of the other homologues) has a valine side chain that would be too small to block the exit in the closed form, if indeed the activation gate is produced by this side chain as has been proposed [1] . This may be because the flexible glycines (its residues 219 and 229) enable a larger hinge motion in the NaChBac S6 helix, placing the polypeptide backbones closer to each other in the closed state. Such sequence differences in S6 may account for the variations in the conductance properties of the bacterial homologues from different species. The availability of crystal structures of prokaryotic homologues of sodium channels with different conformational states of the pore, one in an open conformation (NavMs) and one in a hybrid closed conformation (NavAb), suggests a novel mechanism for channel gating in these channels; it also provides both insight into the nature of the full transmembrane ion pathway and, ultimately, a basis for modelling of ion-translocation events in this physiologically important class of ion channels. The differences between the open and closed structures lie primarily in the C-terminal end of the S6 helix. A simple rotation of the backbone at Thr209, insufficient to disrupt the helical structure, produces a movement of the lower end of the helix away from the pore axis, splaying the cytoplasmic mouth of the channel, and considerably opening up the translocation pathway. This relatively simple mechanism is different from the twisting motion proposed for potassium channels and nicotinic acetylcholine receptors, and from the iris mechanism that has been proposed by analogy, for sodium channels. Thus, this structure is expected to transform our current ideas of gating in homologues of sodium channels. Protein purification The sodium channel pore construct from Magnetococcus sp. (strain MC-1), beginning at transmembrane helix 5, was designed based on multiple sequence alignment (ClustalW [16] ) of prokaryotic VGSCs and the MlotiK, Kv1.2–Kv2.1 chimera and KcsA potassium channel crystal structures (PDB codes 3BEH, 2R9R and 1BL8, respectively [17] , [18] , [19] ). It was PCR-amplified to incorporate an N-terminal Nde I (underlined) and a C-terminal Bam HI site (underlined) using the forward primer, 5′-GCTCTTGGCA CATATG GGCGTGGGCTCG-3′, and the reverse primer, 5′-AGCAGCC GGATCC TTAATGGTG-3′. The PCR product was digested with Nde I and Bam HI, and ligated into pET15b. It was overexpressed in C41(DE3) cells upon addition of 0.5 mM isopropylthiogalactoside at A 600 nm 0.8 for 3.5 h at 37 °C. Cell pellets were suspended in 20 mM Tris, pH 7.5, supplemented with 0.2 mM phenylmethanesulphonyl fluoride, 2 μg ml −1 DNase I and 2.5 mM MgSO 4 , and lysed by cell disruption using an Avestin EmylsiFlex-C5. The lysate was centrifuged at 10,000 g for 30 min to pellet unlysed cells. The supernatant was centrifuged at 43,000 g for 1 h to pellet membranes. Membranes isolated from 12 l culture were solubilized in 100-ml 20 mM Tris, pH 7.5, 300 mM NaCl, 20 mM imidazole and 1% n-dodecyl-β- D -maltopyranoside (SOLGRADE, Affymetrix) for at least 2 h, and loaded onto a 1-ml HisTrap HP (GE Healthcare), using a peristaltic pump, and recirculated overnight at 4 °C. The column was connected to an AKTA FPLC and washed with 20 mM Tris–HCl, pH 7.5, 300 mM NaCl, 20 mM imidazole and 0.52% HEGA-10 (ANAGRADE, Affymetrix) or 0.56% n-nonyl-β- D -maltopyramoside (NM) (ANAGRADE, Affymetrix). The protein was eluted using a 20-column volume gradient of 20 to 500 mM imidazole, and concentrated using a 50 kDa cutoff Amicon Ultracentrifugal filter. The imidazole was exchanged by concentration/dilution before thrombin cleavage. Thrombin cleavage took place at 18 °C for 36 h at 20 units per 4 mg of protein. The mixture was loaded onto a 2 ml HisTrap HP (GE Healthcare) in 25 mM imidazole and the flow-through was collected. It was concentrated to 100 μl before loading onto a gel filtration column (Superdex 200 10/300 GL, GE Healthcare). NavMs pore was eluted with 10 mM Tris–HCl, pH 7.5, 100 mM NaCl and 0.52% HEGA-10 or 0.56% NM at a rate of 0.4 ml min −1 . The pure protein was concentrated to 14 mg ml −1 before setting up crystallizations or frozen at −80 °C. CD spectroscopy The CD spectrum (0.817 mg ml −1 in 10 mM Tris-HCl, pH 7.5, 100 mM NaCl and 0.2% decyl-β- D -maltopyranoside) was collected in a 0.1-mm path-length cell, using an Aviv 62ds spectropolarimeter with a detector acceptance angle of >90° for membrane/scattering samples. Three spectra each of the sample and baseline (all the sample components but without protein present) were collected at 25 °C over the wavelength range from 260 to 185 nm, using a 1-nm step size and a 1-s dwell time. The averaged baseline was subtracted from the averaged sample spectrum, and the spectrum scaled to delta epsilon units using a mean residue weight of 110.96 Da. Data processing used CDtools software [20] . Secondary structure analysis was performed using the DichroWeb server [21] with the CONTINLL algorithm [22] and the SP175t reference data set [23] . Sodium flux uptake and channel-blocker inhibition Experiments with full length and pore constructs of NavMs were performed as previously described for the NavSp homologue [2] . Protein (20–30 μg) was added to 100 μl of lipid (1 mg) 3:1 POPE (1-palmitoyl-2-oleoyl-3-phosphatidylethanolamine) and POPG (1-palmitoyl-2-oleoyl-sn-glycero-3-phospho-(1′-rac-glycerol)) (Avanti Polar Lipids, Inc.) solubilized in buffer A (450 mM NaCl, 10 mM HEPES, 4 mM NMG ( N -methyl-d-glucamine), 1 mM EDTA, pH 7.5) and incubated for 30 min. Liposomes were formed by adding the protein/lipid sample to partially dehydrated Sephadex G-50 columns presoaked in buffer A through polystyrene columns (Pierce Chemical, Co.) and spinning to 2,500 r.p.m. The extra-liposomal solution was exchanged by spinning the sample to 2,500 r.p.m. through a second set of partially dehydrated columns, now containing beads soaked in buffer B (400 mM sorbitol, 10 mM HEPES, 4 mM NMG, 1 mM EDTA, pH 7.5). Uptake of 22 Na + was initiated by adding 400 μl of buffer B containing 22 Na + and the indicated concentration of mibefradil. At various time points, 60 μl aliquots were flowed through 0.5 ml Dowex cation-exchange columns charged with NMGH + to remove extraliposomal 22 Na + . These aliquots were then mixed with scintillation fluid and counted in a liquid scintillation counter. Fractional flux at 60 min in the presence of mibefradil was determined at each time point following subtraction of counts measured for protein-free liposomes. Crystallization/data collection Crystals were grown at 4 °C using the vapour-diffusion method. The NM-solubilized protein was mixed in a 1:1 ratio with reservoir solution containing 0.1 M NaCl, 0.1 M MOPS, pH 7.0, and 30% PEG400 for 200 nl sitting drops, and the HEGA-10-solubilized protein was mixed in a 2:1 ratio with reservoir solution containing 0.09 M tri-sodium citrate, pH 5.6, 30% v/v PEG400 for 3 μl hanging drops. Crystals appeared by 2 days and reached a maximum size of 200 × 200 × 300 μm after 5–7 days. The best of the NM crystals diffracted to 4.2 Å resolution, and the best of the HEGA-10 crystals diffracted to ~4.0 Å resolution. To improve the resolution, an “in house” dehydration method was used: The crystal was mounted onto a cryo-loop, and a yellow tip containing 20 μl of a saturated ammonium chloride solution at its sealed tip was drawn over it and incubated for 16 h at 4 °C. The best of these HEGA-10 crystals showed maximal diffraction to 3.49 Å. The crystals were cryo-cooled and screened using the Birkbeck ‘in house’ X-ray facility, Diamond Light Source, Swiss Light Source and European Synchrotron Radiation Facility. More than 2,000 crystals were screened from over 200 conditions. The data collection and processing statistics are listed in Table 1 . Structure determination The space group of the 3.49 Å HEGA-10 crystals was C121 with cell parameters of 117.1, 74.1, 107.9 (90, 118.3, 90); the data was integrated and scaled using XDS [24] . The symmetry suggested one tetramer per asymmetric unit with a solvent content of 69.3%. The space group of the NM crystals was C2221 with one tetramer in the asymmetric unit and a solvent content of 75.27%. The data were integrated and scaled using iMosflm and SCALA from the CCP4 programme suite [25] . In both cases, the diffraction was anisotropic and a correction was applied using the diffraction anisotropy server [26] . Scaling statistics following anisotropy correction are provided in Table 1 . The structure was solved by molecular replacement with MrBump [27] . The best solution was provided by Phaser [28] , using a search model produced by MOLREP [29] based on the monomer pore region (residue M130 to M221) of the NavAb structure (PDB code 3RVY). Structure building and modification were carried out in COOT [30] and refinement was performed in BUSTER [31] , using the NavAb structure as a high-resolution restraints target, resulting in R/R free of 27.1/28.5%. Although the resolution of the data was only modest, the quality was very high (good statistics and redundancies) and the maps were clear. The crystal packing is mediated by disordered residues and the termini that are not visible in the map, which may explain the limited diffraction quality of many of the crystals. After building the protein chain, there remained strong positive-difference density, in particular at the SF that, given the limited resolution of the data, we were unable to unambiguously model. As we could not be sure that these were sodium ions, we have simply added water molecules at these sites. Refinement quality was checked using the PDB Structure Factor Check software. Structure quality was determined using PROCHECK [32] and MolProbity [33] , which indicated that 100% of the residues were in allowed conformations. The symmetric tetramer model was created using Pymol software [13] as follows: NavMs chain A (the one with the largest bend) was separately aligned to chains A, B, C and D from the NavMs structure using the S5 and P-helices, SF and the top of the S6 helix (which were essentially identical in all chains). A similar real-space fit was produced between the A-chain monomer and the respective positions of all four monomers in the lower resolution NM and HEGA-10 structures. Sequence and structure analyses and alignments The sequences of NavMs and the other homologues were aligned with ClustalW [16] and displayed using Jalview software [34] . The secondary structure of NavMs was determined from its crystal structure using the DSSP algorithm [35] as implemented in the 2Struc server [36] , which was also used for the alignment of secondary structural elements of the open and closed channels. Structures were displayed using Pymol software [13] . MOLE software [15] was used to analyse and display the accessible interior diameter of the symmetric pore and APBS software was used to calculate its electrostatic surface [14] . Accession codes: Atomic coordinates and structure factors have been deposited in the Protein Data Bank under accession code 4F4L . Circular dichroism spectra and metadata have been deposited in the Protein Circular Dichroism Data Bank under accession code CD0004012000. The coordinates of the symmetric tetramer model are available from b.wallace@mail.cryst.bbk.ac.uk How to cite this article: McCusker, E.C. et al. Structure of a bacterial voltage-gated sodium channel pore reveals mechanisms of opening and closing. Nat. Commun. 3:1102 doi: 10.1038/ncomms2077 (2012).